Molecular determinants of magnesium-dependent synaptic plasticity at electrical synapses formed by connexin36 Neuronal gap junction (GJ) channels composed of connexin36 (Cx36) play an important role in neuronal synchronization and network dynamics. Here we show that Cx36-containing electrical synapses between inhibitory neurons of the thalamic reticular nucleus are bidirectionally modulated by changes in intracellular free magnesium concentration ([Mg 2+ ] i ). Chimeragenesis demonstrates that the first extracellular loop of Cx36 contains a Mg 2+ -sensitive domain, and site-directed mutagenesis shows that the pore-lining residue D47 is critical in determining high Mg 2+ -sensitivity. Single-channel analysis of Mg 2+ -sensitive chimeras and mutants reveals that [Mg 2+ ] i controls the strength of electrical coupling mostly via gating mechanisms. In addition, asymmetric transjunctional [Mg 2+ ] i induces strong instantaneous rectification, providing a novel mechanism for electrical rectification in homotypic Cx36 GJs. We suggest that Mg 2+ -dependent synaptic plasticity of Cx36-containing electrical synapses could underlie neuronal circuit reconfiguration via changes in brain energy metabolism that affects neuronal levels of intracellular ATP and [Mg 2+ ] i . Magnesium is the second most abundant intracellular cation after potassium, and is a critical cofactor in many enzymatic reactions involving energy metabolism. Magnesium is highly concentrated in cellular organelles, such as mitochondria, nucleus and endoplasmic reticulum, and it binds to several ionic cytoplasmic constituents. Importantly, phosphonucleotides, such as ATP, bind magnesium ions (MgATP 2− ) and the enzymatic hydrolysis of their phosphate groups depends on this interaction [1] . Therefore, the intracellular concentration of free magnesium ([Mg 2+ ] i ) is closely related to cell bioenergetics and is expected to vary according to the state of cellular metabolism and levels of intracellular ATP [2] . Resting [Mg 2+ ] i is less than 10% of total cellular magnesium, and it ranges from 0.2 to 3.5 mM in neurons depending on cell type and species [3] , [4] , [5] . Under physiological conditions, depolarization triggers an increase of [Mg 2+ ] i in sensory neurons [6] , while glutamate exposure induces a [Mg 2+ ] i surge in forebrain and hippocampal neurons [7] , [8] . More recently, it was shown that activation of a nitric oxide signalling pathway can also trigger an increase of [Mg 2+ ] i in hippocampal neurons [9] . Moreover, enhanced [Mg 2+ ] i can be expected with a reduction in the levels of ATP during periods of waking and hyperactivity [10] . Conversely, reduction in [Mg 2+ ] i can be expected with an increase in ATP levels during glucose or lactate exposure [11] and during the first hours of sleep [10] . In pathological conditions, early onset of ischaemic cell death is mainly due to the inability of mitochondria to produce ATP, resulting in the failure to regulate transmembrane ion gradients [12] , which impacts [Mg 2+ ] i . Long-lasting elevation in brain [Mg 2+ ] i occurs in some acute and chronic brain pathologies such as hypoxia/ischaemia [13] , [14] and in patients with schizophrenia [15] . In contrast, [Mg 2+ ] i is reduced after traumatic brain injury [16] , [17] and in patients with Parkinson [18] , Alzheimer [19] , multiple sclerosis [20] , amyotrophic lateral sclerosis [21] , chronic migraine [22] and mitochondrial diseases [23] . Electrical synapses are specialized intercellular junctions formed by clusters of gap junction (GJ) channels that allow bidirectional electrotonic signalling between neurons. Many roles for electrical synapses have been documented, such as synchronization and coordination of neuronal networks [24] , memory formation [25] and lateral excitation in olfactory glomeruli [26] . GJ channels are formed by the connexin (Cx) and innexin gene families in vertebrates and invertebrates, respectively. Six Cx (or innexin) proteins oligomerize into a pore-forming hemichannel (HC), and the docking of two HCs contributed by adjacent cells forms a GJ channel. The docking of HCs from apposing cells containing the same Cx type results in homotypic GJs, while the docking of HCs containing different Cxs results in heterotypic GJs. Sensitivity of junctional conductance ( g j ) to transjunctional voltage ( V j ) is a common property of all GJs. Each apposed/junctional HC (aHC) has two distinct V j -sensitive gates that are responsible for the steady-state g j – V j relationship ( g j,ss – V j ). This relationship is typically symmetric for either polarity of V j in homotypic junctions [27] , but asymmetric in heterotypic junctions where aHCs have V j sensitivity and/or single-channel conductance differences, which leads to an asymmetry in electrical signal transfer and metabolic communication [28] , [29] . An instantaneous g j – V j relationship ( g j,inst – V j ), however, is more relevant with respect to electrical synapses since neuronal membrane potential fluctuates in the ms time scale during action potentials. Many electrical synapses rectify instantaneously [30] , [31] , [32] , [33] ; that is, electrical signals are preferentially transmitted anterogradely or retrogradely. Electrical synapses between neurons in the mammalian central nervous system (CNS) are typically formed by connexin36 (Cx36) [34] , which is commonly expressed throughout the CNS [34] , [35] . Modulation of electrical synapses can occur by different factors such as phosphorylation [36] , [37] , changes in pH [38] and exposure to lipophilic molecules [39] . Interestingly, Cx36-containing electrical synapses can undergo activity-dependent long-term depression [40] or CaMKII- and PKA-dependent long-term potentiation [41] , [42] . We recently reported a novel Mg 2+ -dependent form of electrical synaptic plasticity between neurons of the trigeminal mesencephalic nucleus (MesV) and in heterologous expression systems transfected with Cx36 (ref. 43 ). We showed that the strength of electrical synaptic transmission is augmented or reduced by low or high [Mg 2+ ] i , respectively. The g j of GJs formed of Cxs 26, 30.2, 32, 36, 43, 45, 47 and 57 expressed in HeLa cells was reduced by increasing [Mg 2+ ] i , whereas lowering [Mg 2+ ] i increased g j only in Cx36 expressing cells, indicating that Cx36 GJs are strongly inhibited by normal/resting [Mg 2+ ] i . We also demonstrated that Mg 2+ ions are permeable to Cx36 GJs and an effect of Mg 2+ on g j is fully reversible [43] . Here, we show that electrical synapses formed by Cx36 in the thalamic reticular nucleus (TRN) are also bidirectionally modulated by changes in [Mg 2+ ] i and that an altered Mg–ATP equilibrium can trigger Mg 2+ -dependent plasticity of neuronal electrical coupling. We sought to locate the molecular domains of Cx36 GJ channels that contribute to such unusually high sensitivity to [Mg 2+ ] i using chimeragenesis and site-directed mutagenesis. Our data show that a negatively charged aspartate (D47), located in the first extracellular loop (E1), is responsible for high Mg 2+ -sensitivity. Single-channel analysis of chimeras (CH) reveals that changes in [Mg 2+ ] i affect the voltage-dependent gating of channels without changing the single-channel conductance. We also found that [Mg 2+ ] i modulates the g j,inst – V j dependence of Cx36 GJs by producing a hyperbolic g j,inst – V j relationship that is unique to Cx36 GJs. Previously, we showed that asymmetry in the transjunctional [Mg 2+ ] i results in an asymmetry of steady-state g j ( g j,ss ) dependence on V j (ref. 43 ). We now demonstrate that asymmetry in the transjunctional [Mg 2+ ] i results in an asymmetric g j,inst – V j relationship of homotypic Cx36 GJ channels. Hence, the intercellular gradient of divalent cations, such as Mg 2+ , is a novel mechanism that can generate instantaneous rectification in homotypic Cx36 GJs. In addition, we show that the second extracellular loop (E2) is an important molecular component that contributes to the incompatibility between neuronal Cx36 and astrocytic Cx43 HCs to dock and form functional heterotypic GJs. Electrical synapses in the TRN are modulated by [Mg 2+ ] i To test whether native electrical synapses expressing Cx36 are sensitive to changes in [Mg 2+ ] i , we used a BAC transgenic mouse line (Tg( Gjd2 - EGFP )JM16Gsat/Mmucd) [44] , in which the expression of the enhanced green fluorescent protein (EGFP) reporter gene is driven by the promoter of Cx36 and expression of the endogenous Cx36 protein is left intact. In Gjd2-EGFP mice, one can easily identify EGFP-positive neurons, facilitating the selection of adjacent pairs of electrically coupled neurons for electrophysiological analysis. The TRN was chosen for examination due to its relatively high incidence of electrical coupling [45] . It is a diencephalic layer of GABAergic interneurons that forms a capsule around the ventrobasal complex of the thalamus, and plays an important role in switching states of arousal and consciousness [46] . Acute horizontal slices of mouse thalamus were used for confocal fluorescence imaging of the TRN ( Fig. 1a,b ) and for measuring g j using a dual whole-cell patch clamp ( Fig. 1c ) in pairs of neurons displaying EGFP fluorescence ( Fig. 1d ). From a total of 57 neuronal pairs recorded, 18 pairs were electrically coupled (31.6%). The intrinsic firing properties ( Fig. 1e ) and attenuated evoked responses ( Supplementary Fig. 1 ) of electrically coupled EGFP-expressing neurons were similar to those previously reported [45] . To reduce or increase [Mg 2+ ] i , we used pipette solutions with K 2 ATP or MgATP, respectively, as previously shown [2] , [43] . Pipette solutions with K 2 ATP (7 mM) showed a ~40% increase in g j after 25 min of recording ( Fig. 1f,g ). Conversely, solutions with MgATP (7 mM) showed a ~50% decrease in g j after 25 min of recording ( Fig. 1f,g ). Therefore, inhibitory interneurons from the TRN showed a significant bidirectional Mg 2+ -dependent modulation of g j , in a similar manner as reported for excitatory neurons from the MesV [43] . 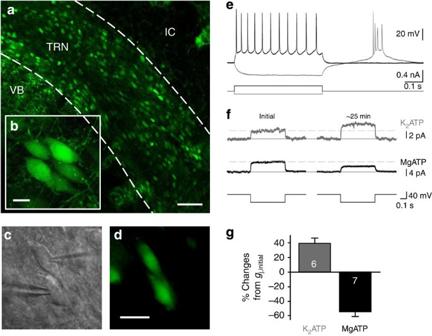Figure 1: Magnesium-dependent plasticity of electrical synaptic transmission between TRN neurons. (a,b) Confocal fluorescence images of horizontal brain slices from a Gjd2-EGFP transgenic mouse showing TRN interneurons expressing EGFP driven by Cx36 promoter. VB, ventrobasal nucleus of the Thalamus; IC, internal capsule. Scale bars correspond to 100 (a) and 10 (b) μm. (c,d) IR-DIC (c) and fluorescence (d) images of an electrically coupled pair of TRN neurons during dual whole-cell patch clamp. Scale bar, 20 μm. (e) Current-clamp recordings from a TRN neuron showing typical spiking and rebound burst behaviour; voltage traces were recorded during 0.5 s current steps of −100 (grey) or 200 pA (black). (f) Voltage-clamp recordings showing averaged transjunctional current traces (10–15 averaged traces) obtained soon after patch openings (initial; left) and after ~25 min of recording (right) for low Mg2+(K2ATP, top) and high Mg2+(MgATP, bottom) conditions; current traces were recorded during 0.5 s transjunctional voltage steps of −40 mV. (g) Mean percentage changes of junctional conductance (gj) from initial values after ~25 min from patch openings with pipette solutions containing 7 mM of K2ATP (grey) or MgATP (black). Numbers of cell pairs are indicated within columns, and error bars correspond to s.e.m. Figure 1: Magnesium-dependent plasticity of electrical synaptic transmission between TRN neurons. ( a , b ) Confocal fluorescence images of horizontal brain slices from a Gjd2-EGFP transgenic mouse showing TRN interneurons expressing EGFP driven by Cx36 promoter. VB, ventrobasal nucleus of the Thalamus; IC, internal capsule. Scale bars correspond to 100 ( a ) and 10 ( b ) μm. ( c , d ) IR-DIC ( c ) and fluorescence ( d ) images of an electrically coupled pair of TRN neurons during dual whole-cell patch clamp. Scale bar, 20 μm. ( e ) Current-clamp recordings from a TRN neuron showing typical spiking and rebound burst behaviour; voltage traces were recorded during 0.5 s current steps of −100 (grey) or 200 pA (black). ( f ) Voltage-clamp recordings showing averaged transjunctional current traces (10–15 averaged traces) obtained soon after patch openings (initial; left) and after ~25 min of recording (right) for low Mg 2+ (K 2 ATP, top) and high Mg 2+ (MgATP, bottom) conditions; current traces were recorded during 0.5 s transjunctional voltage steps of −40 mV. ( g ) Mean percentage changes of junctional conductance ( g j ) from initial values after ~25 min from patch openings with pipette solutions containing 7 mM of K 2 ATP (grey) or MgATP (black). Numbers of cell pairs are indicated within columns, and error bars correspond to s.e.m. Full size image E1 contains a pore-lining Mg 2+ -sensitive domain To locate the position of putative Mg 2+ -sensitive domain/s in Cx36, we performed structure–function studies by assessing g j in response to [Mg 2+ ] i in pairs of RIN cells expressing Cx36/Cx43 CH and mutants with single amino acid substitutions. We selected Cx43 because it shows a higher single-channel conductance ( γ open ; ~110 pS (ref. 47 )), a higher V j -gating sensitivity and a lower sensitivity to changes in [Mg 2+ ] i [43] , relative to Cx36. CH were generated by sequential exchange of corresponding domains of Cx36 and Cx43 using a modified version of the ‘sticky feet’ protocol [48] (See Methods and Supplementary Figs 2 and 3 ). We swapped selected domains at the expected interface between membrane and extracellular domains, and generated a total of sixteen CH from which eight formed junctional plaques (all CH were tagged with EGFP at the C terminus (CT) and expressed in RIN cells) and only four (CH1-CH4) formed functional channels exhibiting electrical cell–cell coupling ( Fig. 2 ). We studied sensitivity to [Mg 2+ ] i by measuring g j at the beginning of the recording ( g j,initial ) and the ratio of g j,final / g j,initial , where g j,final is the g j value at the steady-state level (after ~25 min), using pipette solutions with low or high free Mg 2+ concentrations; [Mg 2+ ] p =0.01 or 5 mM. Cell pairs with approximately the same size of junctional plaques were used to study wild-type and chimeric GJs. The Mg 2+ sensitivity of homotypic GJs formed by CH1 (see Supplementary Fig. 4 for amino acid sequence of functional CH), in which the NT and first transmembrane domain (M1) of Cx36 was replaced by those of Cx43, was similar to the Mg 2+ -sensitivity of Cx36 ( Fig. 3 ). Homotypic GJs formed by CH2 or CH3, in which E1 of Cx43 was replaced by E1 of Cx36, showed Mg 2+ sensitivity similar to that of Cx36 GJs ( Fig. 3 ). GJs formed by CH4, in which only E2 of Cx43 was replaced by E2 of Cx36, showed no changes in sensitivity to Mg 2+ and was similar to that of Cx43 GJs ( Fig. 3 ). Altogether, results from Cx36/Cx43 CH indicate that E1 contains a Mg 2+ -sensitive domain that can be transferred between Cxs, and that NT, M1 and E2 are not involved in Mg 2+ -sensitivity. 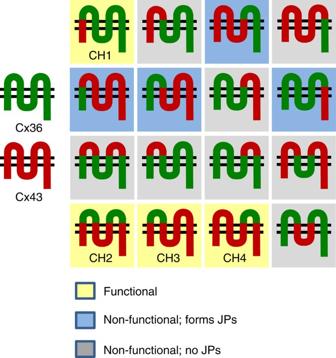Figure 2: All generated Cx36/Cx43 CH. CH were generated from Cx36 (green) and Cx43 (red). CH that form functional channels and junctional plaques (JPs) are shown in yellow background. Functional CH are named from CH1 to CH4. CH that form JPs but do not exhibit electrical cell–cell coupling are shown in blue background. CH that do not form JPs or exhibit electrical cell–cell coupling are shown in grey background. Figure 2: All generated Cx36/Cx43 CH. CH were generated from Cx36 (green) and Cx43 (red). CH that form functional channels and junctional plaques (JPs) are shown in yellow background. Functional CH are named from CH1 to CH4. CH that form JPs but do not exhibit electrical cell–cell coupling are shown in blue background. CH that do not form JPs or exhibit electrical cell–cell coupling are shown in grey background. 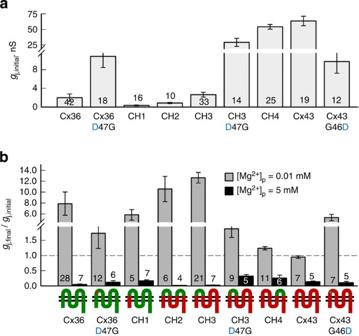Figure 3: Differences in sensitivity to [Mg2+]ibetween Cx36/Cx43 CH and mutants. Experiments were performed in pairs of RIN cells expressing Cx36 (green), Cx43 (red), Cx36/Cx43 CH (CH1-CH4) and amino acid substitutions (D47G or G46D). (a) Mean transjunctional conductance measured soon after patch opening (gj,initial). (b) Meangj(normalized to initialgjvalue) measured after ~25 min using pipette solutions containing 0.01 mM (grey) or 5 mM (black) free Mg2+([Mg2+]p). The dotted line marks the value of normalizedgjequal to 1. Total numbers of cell pairs are indicated within columns, and error bars correspond to s.e.m. Full size image Figure 3: Differences in sensitivity to [Mg 2+ ] i between Cx36/Cx43 CH and mutants. Experiments were performed in pairs of RIN cells expressing Cx36 (green), Cx43 (red), Cx36/Cx43 CH (CH1-CH4) and amino acid substitutions (D47G or G46D). ( a ) Mean transjunctional conductance measured soon after patch opening ( g j,initial ). ( b ) Mean g j (normalized to initial g j value) measured after ~25 min using pipette solutions containing 0.01 mM (grey) or 5 mM (black) free Mg 2+ ([Mg 2+ ] p ). The dotted line marks the value of normalized g j equal to 1. Total numbers of cell pairs are indicated within columns, and error bars correspond to s.e.m. Full size image D47 is critical for determining high sensitivity to [Mg 2+ ] i To locate region/s in E1 that may be responsible for the difference in Mg 2+ sensitivity between Cx36 and Cx43, we generated single amino acid substitutions in non-conserved charged residues of Cx36 and Cx43 ( Supplementary Fig. 5 ). Mutation M52K and V54D in Cx36, and E62N in Cx43 had no effect on Mg 2+ sensitivity. In contrast, GJs formed of Cx36*D47G lost sensitivity to resting/initial [Mg 2+ ] i , while GJs formed of Cx43*G46D gained sensitivity to resting/initial [Mg 2+ ] i ( Fig. 3 ). Position D47 in Cx36 corresponds to position G46 in Cx43. Moreover, GJs formed of CH3*D47G lost sensitivity to resting/initial [Mg 2+ ] i ( Fig. 3 ). In summary, these data demonstrate that E1 contains a Mg 2+ -sensitive domain in which the D47 residue is critical to determine the uniquely high sensitivity of Cx36 GJ channels to Mg 2+ , and that insertion of this single residue in Cx43 confers high sensitivity to Mg 2+ . The γ open of Cx36/Cx43 CH is not affected by [Mg 2+ ] i The γ open of Cx36 GJ channels remains uncertain due to its very low conductance [49] , [50] . For similar reasons, we were unable to examine with sufficient resolution the effects of [Mg 2+ ] i on single Cx36 GJ channels. However, the effect of [Mg 2+ ] i at the single-channel level was amenable to analysis in Cx43-based CH and mutants, which exhibited γ open s similar to that of Cx43 GJs. We found that γ open of CH3 remained unchanged when [Mg 2+ ] p =0.01 and 5 mM ( Fig. 4a,e ). These results are in agreement with our hypothesis that [Mg 2+ ] i controls electrical transmission mostly via gating mechanisms, as we previously suggested using a stochastic 16-state of GJ channels [43] . Furthermore, γ open of homotypic CH3*D47G and CH4 GJs, both with low sensitivity to Mg 2+ compared with that of CH3 GJs, was also similar to γ open of Cx43 and remained unchanged in [Mg 2+ ] p =0.01 and 5 mM ( Fig. 4b,c,e and Supplementary Fig. 6 ). In addition, γ open of Cx43*G46D GJs remained close to that of Cx43 at high and low [Mg 2+ ] p ( Fig. 4d,e ). Homotypic GJs formed by CH3, CH3*D47G, CH4 and Cx43*G46D did not show I j rectification at the single-channel level. Thus, Mg 2+ -dependent changes in g j for these three CH and Cx43 most likely are defined by differences in Mg 2+ -binding affinity and its effects on gating, but not by changes in γ open . 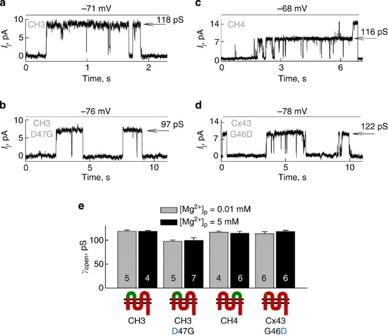Figure 4: Effect of [Mg2+]ion single-channel conductance from homotypic GJs formed by CH3, CH3*D47G, CH4 or Cx43*G46D. (a–d) Transjunctional current (Ij) recordings of single-channel events obtained at indicatedVjs (top) and using [Mg2+]p=0.01 mM. Numbers attached to arrows show single-channel conductances at the open state (γopen). (e) Averagedγopenfor homotypic GJs formed by CH3, CH3*D47G, CH4 and Cx43*G46D using [Mg2+]p=0.01 (grey) or 5 (black) mM. Total numbers of cell pairs are indicated within columns, and error bars correspond to s.e.m. Figure 4: Effect of [Mg 2+ ] i on single-channel conductance from homotypic GJs formed by CH3, CH3*D47G, CH4 or Cx43*G46D. ( a – d ) Transjunctional current ( I j ) recordings of single-channel events obtained at indicated V j s (top) and using [Mg 2+ ] p =0.01 mM. Numbers attached to arrows show single-channel conductances at the open state ( γ open ). ( e ) Averaged γ open for homotypic GJs formed by CH3, CH3*D47G, CH4 and Cx43*G46D using [Mg 2+ ] p =0.01 (grey) or 5 (black) mM. Total numbers of cell pairs are indicated within columns, and error bars correspond to s.e.m. Full size image [Mg 2+ ] i affects g j via gating mechanisms CH3 channels possess the Mg 2+ -sensitive E1 domain of Cx36 ( Figs 2 and 3 ) and the high γ open is similar to that of Cx43 ( Fig. 4 ), which allows for the analysis of Mg 2+ -dependent plasticity at the single-channel level. We studied g j and its dependence on V j in pairs of weakly coupled RIN cells expressing homotypic CH3 GJs. We measured g j,ss – V j relationships using V j ramps from 0 to +90 and −90 mV in amplitude and 30 s in duration ( Fig. 5a , top trace). Under high [Mg 2+ ] p , there was a relatively fast run-down of g j in CH3 GJs, thus g j – V j plots from four consecutive measurements show different g j s at the beginning of each ramp ( Fig. 5a–c ). The initial g j was ~3.8 nS, corresponding to ~33 open CH3 GJ channels ( Fig. 5a,c ). Three minutes later, only one GJ channel was open during the fourth V j ramp (red traces in Fig. 5a,c ). To study the effects of Mg 2+ occupancy inside the pore on V j gating, a transjunctional gradient of [Mg 2+ ] i was created by having different [Mg 2+ ] p ( Fig. 5d ); under these conditions, relative positivity or negativity on the side with higher [Mg 2+ ] i should increase or reduce Mg 2+ occupancy, respectively. The transjunctional asymmetry in [Mg 2+ ] i resulted in strong asymmetric g j,ss – V j dependence measured using V j ramps ( Fig. 5e ). At the single-channel level, negative V j steps applied in the cell with lower [Mg 2+ ] i facilitated closing events, while positive V j steps facilitated opening events ( Fig. 5f ). The γ open of CH3 GJ channels remained at ~115 pS regardless of the V j polarity and Mg 2+ occupancy ( Fig. 5g,h ). These results indicate that an increase in Mg 2+ concentration inside the pore tends to close V j -sensitive gates. 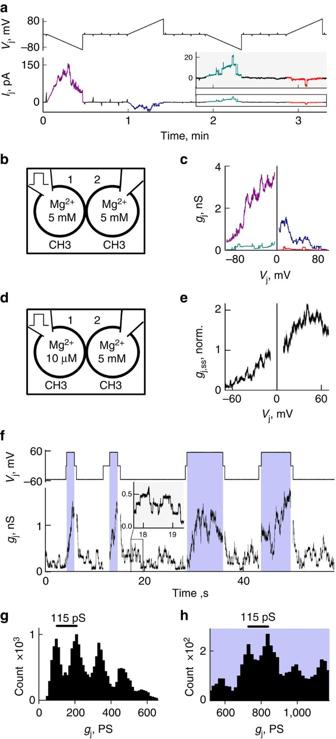Figure 5: Mg2+effect onVjgating and single-channel conductance of homotypic GJs formed of CH3. (a) Changes ofIj(bottom trace) of CH3 GJs in response to repeated 30 s longVjramps from 0 to −90 mV and from 0 to +90 mV with intermediate small amplitude ramps (−10 mV; top trace) using symmetric [Mg2+]p=5 mM. (b,d) Diagrams illustrating [Mg2+]pin cell-1 and cell-2 and the stimulation site of theVjprotocol for experiments shown inaandc(b) ore(d). (c)gj–Vjrelations obtained from experiment shown ina. Colours match theIjdata shown ina. (e) Asymmetricgj,ss–Vjdependence (normalized togjvalue atVjzero) was measured by applyingVjramps from 0 to −70 and from 0 to +70 mV (30 s in duration) under transjunctional Mg2+asymmetry shown ind. Negative potentials applied on the side with low [Mg2+]idecreasedgjpresumably by increasing Mg2+occupancy of the pore through ionophoresis (n=4). (f)gjtrace (bottom) showing unitary gating events of the homotypic CH3 GJ channel obtained duringVjsteps of ±55 mV (top trace) applied in cell-1 (as illustrated ind). NegativeVjs facilitated closing transitions, whereas positiveVjs facilitated opening transitions. (g–h) Count histograms for allgjdata obtained at negative (g) or positive (h)Vjs shown in (f). Both histograms show peaks corresponding to the single-channel conductance of ~115 pS. Figure 5: Mg 2+ effect on V j gating and single-channel conductance of homotypic GJs formed of CH3. ( a ) Changes of I j (bottom trace) of CH3 GJs in response to repeated 30 s long V j ramps from 0 to −90 mV and from 0 to +90 mV with intermediate small amplitude ramps (−10 mV; top trace) using symmetric [Mg 2+ ] p =5 mM. ( b , d ) Diagrams illustrating [Mg 2+ ] p in cell-1 and cell-2 and the stimulation site of the V j protocol for experiments shown in a and c ( b ) or e ( d ). ( c ) g j – V j relations obtained from experiment shown in a . Colours match the I j data shown in a . ( e ) Asymmetric g j,ss – V j dependence (normalized to g j value at V j zero) was measured by applying V j ramps from 0 to −70 and from 0 to +70 mV (30 s in duration) under transjunctional Mg 2+ asymmetry shown in d . Negative potentials applied on the side with low [Mg 2+ ] i decreased g j presumably by increasing Mg 2+ occupancy of the pore through ionophoresis ( n =4). ( f ) g j trace (bottom) showing unitary gating events of the homotypic CH3 GJ channel obtained during V j steps of ±55 mV (top trace) applied in cell-1 (as illustrated in d ). Negative V j s facilitated closing transitions, whereas positive V j s facilitated opening transitions. ( g – h ) Count histograms for all g j data obtained at negative ( g ) or positive ( h ) V j s shown in ( f ). Both histograms show peaks corresponding to the single-channel conductance of ~115 pS. Full size image Transjunctional asymmetry of [Mg 2+ ] i induces rectification To determine whether [Mg 2+ ] i affects γ open of Cx36 GJ channels in a V j -dependent manner, we examined the g j,inst – V j relationship at different [Mg 2+ ] i . The g j,inst – V j dependence is relevant to the behaviour of electrical synapses, because V j generated in neurons arises mostly from action potentials with fast (milliseconds) oscillatory changes in the membrane potential. Instantaneous macroscopic I j s ( I j,inst ) mainly reflect the dependence of γ open on V j in the absence of V j -dependent gating. Thus, we measured steady-state and instantaneous g j – V j dependencies at different [Mg 2+ ] i by using different V j protocols ( Fig. 6a,b ). We found that under high [Mg 2+ ] i , the g j,inst (normalized to g j value at zero V j ) of Cx36 GJs increased while the g j,ss decreased by increasing V j s for both polarities ( Fig. 6c , top panel). Low [Mg 2+ ] i fully eliminated or strongly reduced instantaneous and steady-state g j dependencies on V j ( Fig. 6d , top panel). Moreover, transjunctional asymmetry in [Mg 2+ ] i induced asymmetric steady-state and instantaneous g j – V j dependencies ( Fig. 6e , top panel). The effects of symmetric and asymmetric [Mg 2+ ] i on steady-state and instantaneous g j – V j dependencies were still present, albeit reduced, in GJs formed by Cx36*D47G ( Fig. 6c–e , middle panels, & Fig. 6f ), but absent for g j,inst – V j dependence in GJs formed by CH3 ( Fig. 6c–e , bottom panels). In addition, we found that the effects of [Mg 2+ ] i were eliminated in CH1 only for g j,inst – V j but not for g j,ss – V j dependencies ( Supplementary Fig. 7 ), suggesting that residues in NT or M1 of Cx36 are necessary for the peculiar hyperbola-like g j,inst – V j rectification. Altogether, these results suggest that [Mg 2+ ] i affects Cx36 GJ channels by: (1) gating through its binding in E1 and/or stabilizing a closed conformation of the channel; and (2) rectification of I j,inst depending on V j (see Discussion). 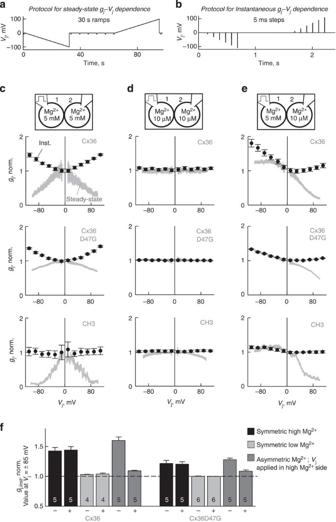Figure 6: GJs formed by Cx36 show Mg2+-dependent rectification of both steady-state and instantaneous conductance–voltage relationships. (a,b)Vjprotocols used to obtain steady-state (a) and instantaneous (b)gj–Vjrelationships. (c–e) Steady-state (grey) and instantaneous (black)gj–Vjrelationships (normalized togjvalue atVjzero) were measured ~30 min after opening of patches under symmetric high (c), low (d), and asymmetric Mg2+conditions (e) in homotypic GJs formed of Cx36 (top row), Cx36*D47G (middle row) and CH3 (bottom row). Each data point for instantaneousgj–Vjrelationships was obtained by averaging data from ~10 consecutiveVjprotocols shown inb, and error bars correspond to s.e.m. Top diagrams in each column show [Mg2+]pand stimulation site. (f) Meangj,instvalues measured atVjs equal to −85 and +85 mV (normalized togj,instvalue atVjzero) at symmetric high (black) and low (light grey) [Mg2+]p, and asymmetric Mg2+conditions (dark grey) for GJs formed of Cx36 (left) and Cx36*D47G (right). Total numbers of cell pairs are indicated within columns, and error bars correspond to s.e.m. Figure 6: GJs formed by Cx36 show Mg 2+ -dependent rectification of both steady-state and instantaneous conductance–voltage relationships. ( a , b ) V j protocols used to obtain steady-state ( a ) and instantaneous ( b ) g j – V j relationships. ( c – e ) Steady-state (grey) and instantaneous (black) g j – V j relationships (normalized to g j value at V j zero) were measured ~30 min after opening of patches under symmetric high ( c ), low ( d ), and asymmetric Mg 2+ conditions ( e ) in homotypic GJs formed of Cx36 (top row), Cx36*D47G (middle row) and CH3 (bottom row). Each data point for instantaneous g j – V j relationships was obtained by averaging data from ~10 consecutive V j protocols shown in b , and error bars correspond to s.e.m. Top diagrams in each column show [Mg 2+ ] p and stimulation site. ( f ) Mean g j,inst values measured at V j s equal to −85 and +85 mV (normalized to g j,inst value at V j zero) at symmetric high (black) and low (light grey) [Mg 2+ ] p , and asymmetric Mg 2+ conditions (dark grey) for GJs formed of Cx36 (left) and Cx36*D47G (right). Total numbers of cell pairs are indicated within columns, and error bars correspond to s.e.m. Full size image Mg 2+ -sensitive heterotypic GJs show asymmetric g j – V j relation Heterotypic GJs formed by Cxs with highly different properties, such as Cx36 and Cx43, present a valuable tool for a high–resolution analysis of the individual aHC properties. Our studies revealed that Cx36 does not form either JPs or functional coupling with Cx43, consistent with reports that neurons and astrocytes do not form Cx36/Cx43 heterotypic GJs [51] . We found that Cx36 or Cx43 were able to form functional heterotypic channels with CH that contain E2 of Cx36 or Cx43, respectively ( Fig. 7 ). Thus, E2 determines incompatibility between Cx36 and Cx43. For heterotypic pairings, we used Cx36 and Cx43 tagged with CFP, while all CH were tagged with EGFP. This allowed us to detect junctional plaques with heterotypic GJs visible in two colours [28] . In Cx43/CH3 heterotypic GJs, both aHCs have a similar unitary conductance ( γ open,H ), but differential sensitivity to [Mg 2+ ] i ( Figs 3 and 4 ). Thus, this heterotypic configuration allows the study of Mg 2+ -sensitivity in CH3 aHCs, and any detected asymmetry can be attributed to the difference in Mg 2+ -sensitivity of aHCs but not γ open,H . Indeed, heterotypic Cx43/CH3 GJs show marked asymmetric g j,ss – V j dependence under symmetric high [Mg 2+ ] i ( Fig. 8a ). At [Mg 2+ ] p =5 mM, positive V j ramps applied on the Cx43 side induced strong gating of the CH3 aHC, suggesting that CH3 aHCs have a negative gating polarity, as has been proposed for Cx43 (ref. 52 ). However, V j -dependent gating of CH3 aHC at negative V j s almost disappears under symmetric low [Mg 2+ ] i ( Fig. 8b ). At the single-channel level, heterotypic Cx43/CH3 GJs showed asymmetric gating behaviour ( Fig. 8c ). Negative V j steps applied on the Cx43 side induced fast flickering of channels, while positive V j steps induced channel closing ( Fig. 8c ). Moreover, the asymmetric gating behaviour of homotypic CH3 GJ channels under asymmetric [Mg 2+ ] i ( Fig. 5c ) can be replicated in heterotypic Cx43/CH3 channels under symmetric [Mg 2+ ] i ( Fig. 8d ). As expected from γ open s of Cx43 and CH3 homotypic GJs, the γ open of heterotypic Cx43/CH3 GJs is ~110 pS, and does not change under high or low [Mg 2+ ] i . Thus, the macroscopic asymmetric g j,ss – V j dependence shown in Fig. 8a can be explained by a Mg 2+ -dependent modulation of gating mechanisms, in which negative potentials induce the transition of gates to a closed state, while positive potentials tend to reopen the gates. At low [Mg 2+ ] i , most of the V j -dependent gating is lost ( Fig. 8b ), suggesting that Mg 2+ is necessary for V j -sensitive gating. Furthermore, we studied g j,ss – V j dependence of Cx43/CH3 GJs under asymmetric [Mg 2+ ] i ( Fig. 8e,f ). These experiments revealed that the direction of the Mg 2+ gradient is important; the g j,ss – V j asymmetry is strengthened when the Cx43 side has higher [Mg 2+ ] i ( Fig. 8e ) or reduced when the Cx43 side has lower [Mg 2+ ] i ( Fig. 8f ). These results strongly support the hypothesis that the site of Mg 2+ interaction in CH3 aHC is located within the pore, and that high [Mg 2+ ] inside the pore increases V j -sensitive gating. 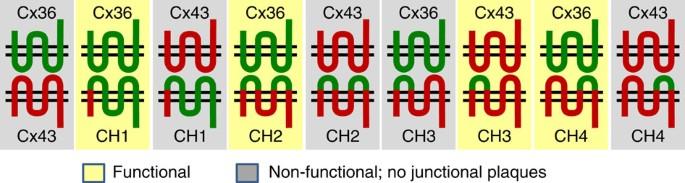Figure 7: Compatibility between Cx36 and Cx43 GJ channels with functional CH. Among all examined heterotypic combinations between wild-type Cx36 (green) or Cx43 (red) with CH1, CH2, CH3 or CH4, only those shown in yellow background formed junctional plaques and exhibit electrical cell–cell coupling, while those shown in grey background did not form junctional plaques or exhibit electrical cell–cell coupling. Figure 7: Compatibility between Cx36 and Cx43 GJ channels with functional CH. Among all examined heterotypic combinations between wild-type Cx36 (green) or Cx43 (red) with CH1, CH2, CH3 or CH4, only those shown in yellow background formed junctional plaques and exhibit electrical cell–cell coupling, while those shown in grey background did not form junctional plaques or exhibit electrical cell–cell coupling. 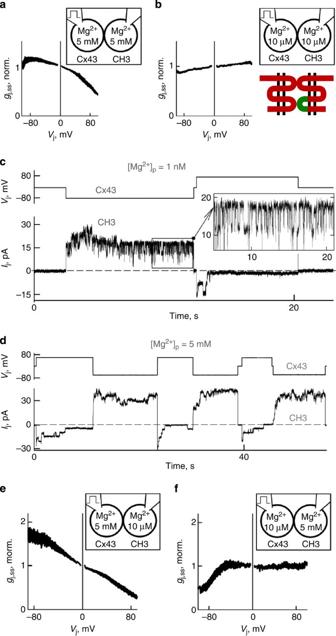Figure 8: Mg2+-dependent asymmetry in steady-stategj–Vjrelationship and single channel conductance in Cx43/CH3 heterotypic GJs. (a,b) Asymmetricgjss–Vjrelationships (normalized togj,ssvalue atVj=0, and obtained using the sameVjprotocol shown inFig. 6a) with pipette solutions containing symmetric high (a) or low (b) [Mg2+]pin heterotypic Cx43/CH3 GJs (n=5). Top diagram in each plot shows [Mg2+]pused in cell-1 and cell-2, stimulation sites and expressed Cxs. (c)Ijrecords of single-channel events at symmetric [Mg2+]pobtained duringVjsteps of ±85 mV (top trace) applied in cell-1 expressing Cx43. (d)Ijrecords (bottom trace) under symmetric high [Mg2+]pshowing unitary gating events of Cx43/CH3 GJ channel obtained duringVjsteps of ±60 mV (top trace) applied in cell-1 expressing Cx43. PositiveVjs facilitated closing transitions, while negativeVjs facilitated opening transitions. (e,f) Asymmetricgjss–Vjrelationships (normalized togj,ssvalue atVj=0) obtained under asymmetric Mg2+conditions (see diagrams) in heterotypic Cx43/CH3 GJs (n=5). Full size image Figure 8: Mg 2+ -dependent asymmetry in steady-state g j – V j relationship and single channel conductance in Cx43/CH3 heterotypic GJs. ( a , b ) Asymmetric g jss – V j relationships (normalized to g j,ss value at V j =0, and obtained using the same V j protocol shown in Fig. 6a ) with pipette solutions containing symmetric high ( a ) or low ( b ) [Mg 2+ ] p in heterotypic Cx43/CH3 GJs ( n =5). Top diagram in each plot shows [Mg 2+ ] p used in cell-1 and cell-2, stimulation sites and expressed Cxs. ( c ) I j records of single-channel events at symmetric [Mg 2+ ] p obtained during V j steps of ±85 mV (top trace) applied in cell-1 expressing Cx43. ( d ) I j records (bottom trace) under symmetric high [Mg 2+ ] p showing unitary gating events of Cx43/CH3 GJ channel obtained during V j steps of ±60 mV (top trace) applied in cell-1 expressing Cx43. Positive V j s facilitated closing transitions, while negative V j s facilitated opening transitions. ( e , f ) Asymmetric g jss – V j relationships (normalized to g j,ss value at V j =0) obtained under asymmetric Mg 2+ conditions (see diagrams) in heterotypic Cx43/CH3 GJs ( n =5). Full size image We studied g j,ss – V j and g j,inst – V j dependencies and sensitivity to [Mg 2+ ] i of Cx36 aHC in Cx36/CH4 heterotypic GJs. This heterotypic configuration allows for a higher resolution analysis of Mg 2+ sensitivity and of V j gating of Cx36 aHCs; in Cx36/CH4 GJs, almost all V j drops across the Cx36 aHCs due to a ~15-fold lower γ open,H than in CH4 (ref. 53 ), making CH4 aHC virtually insensitive to V j . We found that under high symmetric [Mg 2+ ] p (5 mM), g j,inst (normalized to g j value at zero V j ) of heterotypic Cx36/CH4 GJs increased for both polarities of V j ( Fig. 9a , bottom), while g j,ss – V j showed a marked asymmetric dependence ( Fig. 9a , top). Interestingly, g j,inst – V j dependence of heterotypic Cx36/CH4 GJs becomes less symmetric at low [Mg 2+ ] p ( Fig. 9b , bottom), in which g j,inst increased only at relative negativity on the Cx36 side. The asymmetric g j,ss – V j dependence almost disappears under low [Mg 2+ ] p (0.01 mM, Fig. 9b , top) due to a reduction in V j sensitivity, indicating that most of the asymmetry is due to the Mg 2+ sensitivity of Cx36 aHC. To study the mechanism of I j,inst – V j rectification of the Cx36 aHC in more detail, we simulated g j,inst – V j dependence curves that fit our experimental data using a stochastic four state model (S4SM) of GJ channels [54] . g j,inst – V j relationships of the Cx36 homotypic and Cx36/CH4 heterotypic GJs were simulated using a hyperbolic equation describing the Cx36 aHC conductance: γ open,H = γ open,H,0 , where γ open,H,0 is γ open,H at V H =0, V H is voltage across aHC, r H and r Mg are Mg 2+ -independent and Mg 2+ -dependent rectification coefficients of aHC, respectively. The CH4 aHC conductance was described using a single exponential equation: γ open,H = γ open,H,0 . The simulated g j,inst – V j curves for Cx36 (pink) and CH4 (purple) aHCs produced curves with good fit (grey) for steady state and instantaneous g j – V j dependence of experimental data from heterotypic Cx36/CH4 GJs at low and high symmetric [Mg 2+ ] i ( Fig. 9a,b ). The same hyperbolic equation describing γ open,H of Cx36 and similar rectification values used in simulation of heterotypic Cx36/CH4 GJs were also used to simulate experimental data for homotypic Cx36 GJs at high and low [Mg 2+ ] i ( Fig. 9c,d ). All values of rectification and gating parameters are presented in Supplementary Table 1 . 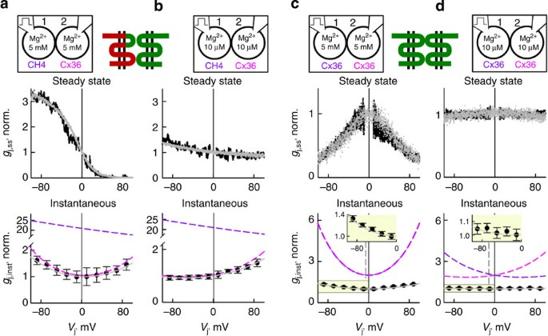Figure 9: Mg2+-dependent asymmetry in steady-state and instantaneousgj–Vjrelationship in Cx36/CH4 heterotypic GJs. (a,b) Asymmetric steady-state (top) and instantaneous (bottom)gj–Vjrelationships shown in black (normalized togjvalue atVj=0, and obtained using the sameVjprotocol shown inFig 6a,b, respectively) obtained under symmetric high (a) and low (b) [Mg2+]pin heterotypic Cx36/CH4 GJs (n=5). The top diagram in each plot shows [Mg2+]pused in cell-1 and cell-2, stimulation sites and expressed Cxs. Each data point forgj,inst–Vjrelationships was obtained by averaging data from ~10 consecutiveVjprotocols, and error bars correspond to s.e.m. Simulated curves shown in grey for steady-state (top) and instantaneous (bottom)gj–Vjrelationships were obtained using the S4SM. Dotted lines showgj,inst–Vjrelationships for CH4 (purple) and Cx36 (pink) aHCs used in simulation of steady-state and instantaneousgj–Vjrelationships. (c,d) Symmetric steady-state (top) and instantaneous (bottom)gj–Vjrelationships for homotypic Cx36 GJs are shown in black (data fromFig. 6c,d). Simulated curves shown in grey were obtained using the S4SM and similar rectification parameters were obtained from Cx36 aHCs shown inaandb. All parameters for simulation are reported inSupplementary Table 1. Figure 9: Mg 2+ -dependent asymmetry in steady-state and instantaneous g j – V j relationship in Cx36/CH4 heterotypic GJs. ( a , b ) Asymmetric steady-state (top) and instantaneous (bottom) g j – V j relationships shown in black (normalized to g j value at V j =0, and obtained using the same V j protocol shown in Fig 6a,b , respectively) obtained under symmetric high ( a ) and low ( b ) [Mg 2+ ] p in heterotypic Cx36/CH4 GJs ( n =5). The top diagram in each plot shows [Mg 2+ ] p used in cell-1 and cell-2, stimulation sites and expressed Cxs. Each data point for g j,inst – V j relationships was obtained by averaging data from ~10 consecutive V j protocols, and error bars correspond to s.e.m. Simulated curves shown in grey for steady-state (top) and instantaneous (bottom) g j – V j relationships were obtained using the S4SM. Dotted lines show g j,inst – V j relationships for CH4 (purple) and Cx36 (pink) aHCs used in simulation of steady-state and instantaneous g j – V j relationships. ( c , d ) Symmetric steady-state (top) and instantaneous (bottom) g j – V j relationships for homotypic Cx36 GJs are shown in black (data from Fig. 6c,d ). Simulated curves shown in grey were obtained using the S4SM and similar rectification parameters were obtained from Cx36 aHCs shown in a and b . All parameters for simulation are reported in Supplementary Table 1 . Full size image Electrical synapses are known to function throughout the mammalian CNS, and Cx36 expression is necessary to produce robust neuronal coupling in many brain areas [35] . We recently showed Mg 2+ -dependent modulation of signal transfer at electrical synapses between excitatory MesV neurons in the midbrain and that this [Mg 2+ ] i effect was similar to that observed in heterologous expression systems [43] . Here, we demonstrated that electrical synapses formed by Cx36 GJs between GABAergic interneurons in the TRN also show Mg 2+ -dependent synaptic plasticity, and that the ratio between the total intracellular ATP and Mg 2+ contributes to regulation of electrical coupling ( Fig. 1 ). Although the magnitude of changes in g j between TRN ( Fig. 1 ) and MesV [43] neurons were significant (~30–40%), they were smaller than those observed in RIN cells expressing Cx36. This distinction may be explained by differences in the initial [Mg 2+ ] i and other divalent cations as well as the concentration of ATP and phosphocreatine, that exert a Mg 2+ buffering capacity, and the location of JPs with respect to patch pipette attachment at the soma. Despite these differences, the magnitude of g j changes is comparable to that of previous reports on long-term depression or potentiation of neuronal coupling [40] , [42] . Taken together, these results support the hypothesis that Mg 2+ -dependent synaptic plasticity of Cx36-containing electrical synapses is neuronal-type independent and is a common mechanism that affects the strength of neuronal electrical coupling in the CNS. We recently suggested that Mg 2+ exerts its effects on g j of Cx36 GJs via interaction with a domain in the channel lumen [43] . This interaction may affect V j -sensitive gates by modulating their sensitivity to voltage and stabilizing a closed state conformation [43] . Previously, we showed that sensitivity to high [Mg 2+ ] i is similar in wild-type Cx36 and Cx43, and tagged with fluorescent proteins [43] . Here, using colour variants of GFP tagged to Cx36/Cx43 CH and mutants, we demonstrate that E1 of Cx36 contains a Mg 2+ -sensitive domain and that it can be transferred to Cx43 ( Fig. 3 ). In addition, single amino acid substitutions targeted to E1 of Cx36 and Cx43 revealed that residues in E1 are indeed responsible for the sensitivity to Mg 2+ and that particularly D47 is critical for high Mg 2+ sensitivity in Cx36 GJs ( Fig. 3 ). Interestingly, the G46D mutation in Cx43 (corresponding location of D47 in Cx36) was sufficient to significantly increase sensitivity to Mg 2+ in Cx43 ( Fig. 3 ). Furthermore, as predicted from the crystal structure of Cx26 (ref. 55 ), the side chains of the residue D47 in GJs formed by Cx36 face the pore, form a negatively charged hexameric ring and contribute significantly to the negative surface potential of the pore ( Fig. 10a–c ), supporting the view that Mg 2+ interacts with a pore-lining domain located in E1 and that residue D47 provides strong electro negative surface potential, which may increase Mg 2+ occupancy. It is noteworthy that recent quantum chemistry studies in Cx26 structure have proposed that Ca 2+ may directly interact with E47 (E49 in Cx36) to induce closure of the channel by a gating mechanism [56] . Other intracellular cations, such as spermine, have been shown to affect V j -dependent gating mechanisms by interacting with charged residues located in the N terminus [57] . In addition, spermine can influence the Mg–ATP binding affinity [2] , and therefore modulate its action on g j and gating. 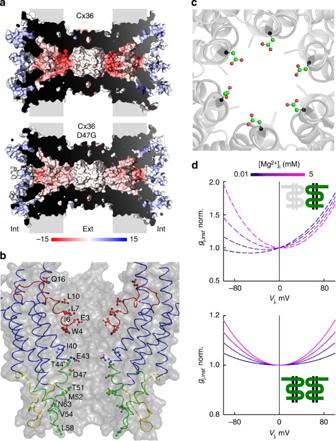Figure 10: Homology models of Cx36 and Cx36*D47G GJ channel structure and Mg2+-dependent modulation of instantaneous rectification. (a) Cross-sections of GJ channels formed by Cx36 (top) or Cx36*D47G (bottom) generated by sequence homology to Cx26 crystal structure. Electrostatic surface potential is displayed for both channels and was estimated with DELPHI (see Methods). The colour bar at the bottom represents electrostatic surface potentials ranging from −15 (red) to 15 (blue)kTe−1. (b) Side view of a Cx36 aHC indicating the pore-lining residues of only two Cx subunits represented with thin ribbon style (principal chain). Main domains of Cx subunits are depicted with different colours and the side chains of pore-lining residues are represented with sticks and spheres. (c) View of the pore from the centre of the channel towards the cytoplasmic mouth. The six D47 residues are displayed with sticks and spheres to illustrate the orientation and position of their side chains with respect to the lumen of the channel. (d) Normalizedgj,inst–Vjplots for aHCs (top) and GJ channels (bottom) formed by Cx36 generated using different values for Mg2+-dependent coefficient (rMg) with the S4SM of GJ channels gating. Colour bar at the top represents different [Mg2+]ifrom 0.01 to 5 mM. Figure 10: Homology models of Cx36 and Cx36*D47G GJ channel structure and Mg 2+ -dependent modulation of instantaneous rectification. ( a ) Cross-sections of GJ channels formed by Cx36 (top) or Cx36*D47G (bottom) generated by sequence homology to Cx26 crystal structure. Electrostatic surface potential is displayed for both channels and was estimated with DELPHI (see Methods). The colour bar at the bottom represents electrostatic surface potentials ranging from −15 (red) to 15 (blue) kTe − 1 . ( b ) Side view of a Cx36 aHC indicating the pore-lining residues of only two Cx subunits represented with thin ribbon style (principal chain). Main domains of Cx subunits are depicted with different colours and the side chains of pore-lining residues are represented with sticks and spheres. ( c ) View of the pore from the centre of the channel towards the cytoplasmic mouth. The six D47 residues are displayed with sticks and spheres to illustrate the orientation and position of their side chains with respect to the lumen of the channel. ( d ) Normalized g j,inst – V j plots for aHCs (top) and GJ channels (bottom) formed by Cx36 generated using different values for Mg 2+ -dependent coefficient ( r Mg ) with the S4SM of GJ channels gating. Colour bar at the top represents different [Mg 2+ ] i from 0.01 to 5 mM. Full size image Single-channel analysis of Cx43-based CH and mutants (CH2, CH3, CH4 and Cx43*G46D) showed that γ open is not affected by [Mg 2+ ] i ( Fig. 4 ), and a long-lived residual state is absent, indicating that the fast gating mechanism is inhibited most likely due to C terminus tagging by fluorescent proteins [58] . The latter can reduce g j,ss dependence on V j in Cx43/CH3 heterotypic GJs ( Fig. 8 ), but should not influence g j,ss – V j dependence of Cx36/CH4 GJs ( Fig. 9 ) due to a significant difference in γ open,H of Cx36 and CH4 aHCs, making CH4 aHC unlikely to be gated by V j . In addition, γ open and V j -sensitive gating records under transjunctional asymmetry in [Mg 2+ ] i allowed us to conclude that changes in [Mg 2+ ] inside the pore are necessary for the observed asymmetry in the g j,ss – V j relationship of CH3 GJs ( Figs 5d–f and 8e,f ). Cx36 is not compatible to dock with Cx43, but is compatible with CH2 and CH4. Cx43 is compatible with CH1 and CH3 but not with CH2 and CH4 ( Fig. 7 ). These data suggest that E2 is an important structural determinant for the incompatibility between Cx36 and Cx43, consistent with reports showing the key role E2 plays in determining compatibility between different Cxs [59] , [60] . Cx43/CH3 heterotypic GJs showed a marked asymmetry in the g j – V j relationship, and this asymmetry was dependent on [Mg 2+ ] i ( Fig. 8a,b ). CH3 GJs exhibited similar sensitivity to Mg 2+ compared with that of Cx36 ( Fig. 3 ), while its γ open is >15-fold higher than that of Cx36. Macroscopic and single-channel recordings of Cx43/CH3 GJs ( Fig. 8a,d ) under high [Mg 2+ ] i show significant V j gating asymmetry with pronounced sensitivity to V j at relative negativity on the CH3 side. The dependence of V j gating asymmetry on the Mg 2+ gradient in Cx43/CH3 heterotypic GJs ( Fig. 8e,f ) demonstrates that asymmetric gating is determined not only by [Mg 2+ ] i concentration inside the pore, but also by its influence on V j sensitivity. When [Mg 2+ ] i is higher on the Cx43 side, the g j,ss – V j asymmetry is enhanced compared to that under high symmetric [Mg 2+ ] i . These effects are presumably due to increased V j gating and Mg 2+ occupancy during positive V j s applied on the Cx43 side, and decreased V j gating and Mg 2+ occupancy during negative V j s applied on the Cx43 side ( Fig. 8e ). Conversely, when [Mg 2+ ] i is lower on the Cx43 side, the g j – V j asymmetry is reduced and opposite compared with the one at high symmetric [Mg 2+ ] i ( Fig. 8f ). Consistent with our data, a three-state model of Mg 2+ -dependent gating of Cx37 HCs, also suggests the stabilization of a closed state by Mg 2+ binding [61] . We found a unique g j,inst – V j relationship dependence on [Mg 2+ ] i of Cx36 GJ channels. Reported and preliminary data show that all examined Cxs with the exception of Cx36 demonstrate no or minimal decay of g j,inst dependence on V j for both V j polarities [52] . The symmetric increase in g j,inst at high V j s for Cx36 was previously reported in the oocyte expression system at normal/resting [Mg 2+ ] i [62] . Here, we show that g j,inst s at high [Mg 2+ ] i increases ~1.4 fold at V j =±100 mV, and that this increase disappears under low [Mg 2+ ] i ( Fig. 6c,d ). All our attempts to replicate the observed g j,inst – V j dependence at high [Mg 2+ ] i using a one-dimensional Poisson–Nernst–Plank model [63] were unsuccessful. Studies of heterotypic CH4/Cx36 GJs show that g j,inst increased for both polarities of V j at high [Mg 2+ ] i ( Fig. 9a ) and only at relative negativity of V j at low [Mg 2+ ] i on the Cx36 side ( Fig. 9b ). Thus, the g j,inst – V j relationship of Cx36 aHC transforms from hyperbola-like to exponential-like when [Mg 2+ ] p decreases from 5 to 0.01 mM ( Fig. 9a,b ). An approximately 15-fold difference in γ open,H between Cx36 and CH4 aHCs allows us to assume that measured g j,inst – V j rectification in Cx36/CH4 GJs can be attributed solely to the Cx36 aHC. These data suggest that g j,inst – V j rectification of Cx36 aHC contains two exponential-like components in opposite orientation with respect to V j polarity, defined by: (1) asymmetry of fixed charges inside the Cx36 aHC pore, as described by Poisson–Nernst–Plank equations [63] ; and (2) [Mg 2+ ] i . Figure 10d (top) shows a family of simulated g j,inst – V j plots for Cx36 aHCs using S4SM (details in the Results section), in which the rectification coefficient, r H , was constant and equal to 90 mV, and the Mg 2+ -dependent rectification coefficient, r Mg , changed from ~200 to 80 mV when [Mg 2+ ] i increased from ~0.01 to 5 mM. Figure 10d (bottom) shows simulated g j,inst – V j plots of homotypic Cx36 GJs using the same parameters as for Cx36 aHCs. Thus, Mg 2+ -dependent rectification can explain the transformation of g j,inst – V j dependence observed in heterotypic Cx36/CH4 ( Fig. 9a,b ) and homotypic Cx36 ( Fig. 9c,d ) GJs. Hyperbola-like conductance–voltage rectification has also been shown in a solid back-to-back p–n junction [64] , but applicability of such junctions to GJ channels remains unclear. The g j,inst – V j rectification was not observed under high or low [Mg 2+ ] i in CH1 GJs ( Supplementary Fig. 7 ), suggesting that residues in the NT-M1 region of the Cx36 protein are necessary for instantaneous rectification. To our knowledge, molecular mechanisms of electrical rectification in GJs have been examined only in heterotypic GJs. In this regard, two mechanisms have been proposed: differences in fast V j -dependent gating and gating polarity of aHCs of heterotypic GJs [65] , [66] ; and/or rectification of the single-channel conductance resulting from an asymmetry in the number and position of charged residues inside the channel pore of heterotypic GJs [67] . Thus, we propose that transjunctional asymmetry in [Mg 2+ ] i can serve as a novel mechanism for electrical rectification in homotypic GJs ( Fig. 6e ). It is important to note that the degree of rectification in electrical synapses has been proposed to affect the dynamic output of neuronal networks [68] , and therefore this novel instantaneous Mg 2+ -dependent rectification could be important to explain the phenomenon of switching between firing states and changes in the output of neuronal networks during different metabolic states where [Mg 2+ ] i is affected. Taken together, these findings suggest that changes in [Mg 2+ ] i may be sufficient to induce plasticity of Cx36-based electrical synaptic transmission. Generation of CH and mutants All CH were generated using a modified version of the ‘sticky feet’–directed mutagenesis protocol [48] . Briefly, long PCR oligonucleotide primers that share a complementary sequence were used as forward or reverse primers to isolate fragments with complementary ends of two different genes (1st PCR step). Subsequently, these long DNA fragments were used as primer DNAs to produce chimeric fragments from two different genes (2nd PCR step). This protocol is illustrated in Supplementary Fig. 2 . A total of 22 different DNA fragments with complementary ends (FX-1 and FX-2) were generated to produce 14 different chimeric fragments (FX; Supplementary Fig. 3 ). Two additional chimeric fragments (F12 and F16) were generated by restriction enzyme subcloning ( Supplementary Fig. 3 ). A list of all primer sequences and restriction enzymes used in the generation of each DNA fragment is provided in Supplementary Table 2 . Design of primers was assisted by Clone Manager Professional 9 (Sci-Ed software, NC, USA). Platinum PCR SuperMix High Fidelity (Life Technologies, NY, USA) were used for all PCRs. PCR products were separated by acrylamide gel electrophoresis and isolated with a gel extraction kit (Qiagen). All restriction enzymes were purchased from New England Biolabs. Amino acid substitutions in Cx36 and Cx43 were introduced using the Quickchange Multi Site-directed Mutagenesis Kit (Agilent, TX, USA) or ordered from Genscript (New Jersey, USA) using the site-directed mutagenesis service. CH and mutant fragments were subcloned into pEGFP-N1 (Clontech, CA, USA). All plasmid transfections were performed with Lipofectamine 2000 (Life Technologies, NY USA). Cell lines and culture conditions Experiments were performed in RIN cells (rat beta-cell insulinoma, ATCC CRL-2057) transfected with Cx36, Cx43, CH or mutants fused with colour variants of green fluorescent proteins (EGFP or CFP) attached to the CT. All experiments were performed with stable cell lines to minimize variability. All cell cultures were grown in RPMI 1640, with L -glutamine, supplemented with 8% fetal calf serum, 100 μg per ml streptomycin and 100 units per ml penicillin, and maintained in a CO 2 incubator (37 °C and 5% CO 2 ). In vitro electrophysiology Electrophysiological recordings were performed in cell cultures grown on glass coverslips and submerged on an experimental chamber mounted on the stage of an inverted IX70 microscope (Olympus) equipped with a fluorescence imaging system. Extracellular solution contained (in mM): 140 NaCl, 4 KCl, 2 CaCl 2 , 1 MgCl 2 , 2 CsCl, 1 BaCl 2 , 5 glucose, 2 pyruvate and 5 HEPES (pH 7.4 adjusted with NaOH). Standard pipette solution contained (in mM): 130 CsCl, 10 NaAsp, 1 MgCl 2 , 0.26 CaCl 2 , 2 EGTA and 5 HEPES (pH 7.2 adjusted with CsOH). Resistance of recording pipettes was in the order of 3–5 MΩ. We used either EDTA or MgCl 2 and the web-based Maxchelator software to adjust and calculate free Mg 2+ concentration in the pipette solutions. Junctional conductance ( g j ) was measured using two EPC-8 patch clamp amplifiers (HEKA); briefly, a transjunctional voltage ( V j ) was generated by modifying voltage in cell-1 ( V 1 ) and keeping the voltage in cell-2 ( V 2 ) constant ( V j =Δ V 1 ). Application of V j induced a transjunctional current ( I j ) of opposite polarity to V j ( I j =−Δ I 2 , and g j = I j / V j ). Signals were digitized using an A/D converter (Axon instruments) and data were acquired and analysed using custom-made software. Brain-slice preparation and electrophysiology A minimal number of animals were killed in accordance with the National Institute of Health Guide for the Care and Use of Laboratory Animals , and with the provisions of the Institutional Animal Care and Use Committee of the Marine Biological Laboratory. Horizontal brain slices (300-μm thick) were prepared from the BAC transgenic mouse line Tg( Gjd2 - EGFP )JM16Gsat/Mmucd [44] , in which the expression of EGFP reporter gene is driven by the activity of the Cx36 promoter. Male or female mice age between P5 and P15 were used. Brain slices were obtained using a chilled VT1200 blade vibrating microtome (Leica Biosystems, IL, USA) and sliced in cold sucrose solution containing (in mM): 238 sucrose, 2.7 KCl, 1.25 KH 2 PO 4 , 26 NaHCO 3 , 11 Glucose, 2 CaCl 2 and 2 MgSO 4 . Brain slices were transferred to an incubation chamber with extracellular recording solution and incubated for 20 min at 37 °C. The extracellular recording solution contained (in mM): 124 NaCl, 2.7 KCl, 1.25 KH 2 PO 4 , 26 NaHCO 3 , 10 Glucose, 2 CaCl 2 and 2 MgSO 4 . The incubation chamber was then kept at room temperature for 30–40 min before electrophysiology. Brain slices were then transferred to a low-noise RC-27LD recording chamber (Warner Instruments, Hamden, CT) mounted on an Axio Examiner A1 microscope (Zeiss, Thornwood, NY) equipped with an Orca-R2 digital camera (Hamamatsu, Bridgewater, NJ) for infrared differential interference contrast (IR-DIC) and fluorescence imaging. Extracellular recording solution was continuously exchanged (~2 ml per min) at room temperature in the chamber by a gravity feed perfusion system. All sucrose and extracellular solutions were constantly bubbled and saturated with carbogen (95% oxygen/5% CO 2 ) throughout the slice procedure and electrophysiology experiments. TRN neurons were identified based on characteristic location, cell shape and electrophysiological properties [45] . A standard pipette solution contained (in mM): 120K-Gluconate, 20 KCl, 2 MgCl 2 , 0.2 EGTA, and 10 HEPES (pH 7.2 adjusted with KOH). Resistance of recording pipettes was on the order of 6–10 MΩ. We used K 2 ATP or MgATP to decrease or increase, respectively, free Mg 2+ concentration in the pipette solutions [2] , [43] . Changes in membrane voltage and current were measured using two separate Axopatch 200B amplifiers, digitized using a Digidata 1,440A, and acquired and analysed using pClamp 10 software (Molecular Devices, Sunnyvale, CA). The g j was measured and calculated as explained for the in vitro electrophysiology (see above). Confocal microscopy and fluorescence imaging Fluorescence signals from EGFP expression in acute TRN brain slices were acquired using a LSM-780 Quasar confocal system configured on an inverted Observer Z1 microscope. Imaging during electrophysiology studies was conducted using an Axio Examiner A1 microscope (Zeiss, Oberkochen, Germany) equipped with an Orca-R2 digital camera (Hamamatsu Corp., Bridgewater, NJ). Image acquisition and processing were performed using ZEN software (Zeiss, Oberkochen, Germany). For in vitro studies, fluorescence signals from EGFP or CFP were acquired using an IX70 microscope (Olympus, USA) equipped with an ORCA-R2 digital camera (Hamamatsu Corp., Bridgewater, NJ). Image acquisition and processing were performed using UltraVIEW software (Perkin Elmer Life Sciences, Boston, MA). Homology models and electrostatic surface potential Structural homology models of Cx36 and Cx36*D47G were built using the known three-dimensional structure of Cx26 as a template [55] . The corresponding Cx26 cytoplasmic loop and C terminus domains of Cx36 were deleted, and the target-template alignment was selected by hand, scoring a sequence identity of 47%. On the basis of this alignment, 200 models were generated by means of the MODELLER program and the best model was selected according to the DOPE score [69] . The electrostatic potential on the solvent accessible surface (surface potential) of the structural homology models was estimated using DELPHI, which provides finite difference solutions to the Poisson-Boltzmann equation [70] . Surface potentials are displayed according to the averaged electrostatic potential found at the surface of the Cx accesible to the solvent. Default dielectric constants of 2.0 for interior (protein) and 80.0 for exterior (solvent) regions were used. Data analysis The analysis and statistics were performed using SigmaPlot v10 (Systat Software Inc, Chicago, IL) and pClamp 10 (Molecular Devices). Averaged data are reported as the means±s.e.m. Means for each group were compared using an unpaired Student’s t -test. How to cite this article: Palacios-Prado, N. et al. Molecular determinants of magnesium-dependent synaptic plasticity at electrical synapses formed by connexin36. Nat. Commun. 5:4667 doi: 10.1038/ncomms5667 (2014).